Reprogramming to pluripotency is an ancient trait of vertebrate Oct4 and Pou2 proteins The evolutionary origins of the gene network underlying cellular pluripotency, a central theme in developmental biology, have yet to be elucidated. In mammals, Oct4 is a factor crucial in the reprogramming of differentiated cells into induced pluripotent stem cells. The Oct4 and Pou2 genes evolved from a POU class V gene ancestor, but it is unknown whether pluripotency induced by Oct4 gene activity is a feature specific to mammals or was already present in ancestral vertebrates. Here we report that different vertebrate Pou2 and Oct4 homologues can induce pluripotency in mouse and human fibroblasts and that the inability of zebrafish Pou2 to establish pluripotency is not representative of all Pou2 genes, as medaka Pou2 and axolotl Pou2 are able to reprogram somatic cells into pluripotent cells. Therefore, our results indicate that induction of pluripotency is not a feature specific to mammals, but existed in the Oct4/Pou2 common ancestral vertebrate. The evolution of the network of transcription factors responsible for not only inducing but also maintaining pluripotency is receiving widespread attention from the scientific community. The transcription factor Oct4 (ref. 1 ) is considered to be a key factor in this pluripotency network, as it is required for the maintenance of a pluripotent cell state in the early embryo [2] and in embryonic stem cells (ESCs) derived therefrom [1] , [3] . Oct4 as well as Pou2 genes are members of the Class V POU family [4] . Oct4 was first suggested to have arisen by duplication of the Pou2 gene during the evolution of the early mammal [5] . A subsequent analysis concluded that the gene may have duplicated earlier in the tetrapod lineage [5] . Marsupial (for example, platypus and tammar) and monotreme (for example, opossum) mammals have retained both genes, whereas other vertebrates have retained only one of the two family members [4] , [5] . On the basis of sequence homology, actinopterygii (for example, zebrafish and medaka), aves (for example, chicken) and amphibia from the anura order (for example, frog) have all retained Pou2 , whereas amphibia from the caudata order (for example, axolotl), reptilian (for example, lizard) and eutherian (for example, mouse and human) mammals have retained Oct4 (refs. 4 , 6 ). Interestingly, this pattern of gene retention correlates with the divergent mechanisms of germ cell formation found among vertebrates. Fish, frog and chicken that retained Pou2 present a determinative germ cell formation, meaning that germ cells form through the segregation of germ plasm. In contrast, axolotl and mammals that retained Oct4 present an inductive germ cell formation, meaning that germ cells are formed via induction of embryonic mesoderm [7] , [8] . Furthermore, Pou2 is considered to be weakly associated with the pluripotent cell state, as it is also expressed in somatic tissues such as the brain, whereas Oct4 is exclusively expressed in pluripotent cells and germ cells. Studies examining the ability of different vertebrate Oct4 / Pou2- like homologues to replace endogenous Oct4 in mouse ESCs indicated that xenopus Oct91 and chicken cPouV orthologs could significantly rescue pluripotency in Oct4 -deficient mouse ESCs. In contrast, the zebrafish Pou2 ortholog had little if any rescuing ability, suggesting variability in pluripotency-sustaining activity between the Oct4 and Pou2 genes [5] , [9] , [10] . In order to bind to target gene promoters, the OCT4 –SOX2 protein complex cooperatively assembles to DNA sequences containing a specific arrangement of the Oct4 and Sox2 binding sites [11] . Through such dimers, OCT4 and SOX2 bind together to many promoters of pluripotency-associated genes [12] and orchestrate the pluripotency network [13] . The exogenous overexpression of Oct4 and Sox2 is essential for inducing the reprogramming of somatic cells to a pluripotent cell state, and excluding one or the other transcriptional factor from the reprogramming cocktail completely abolishes the generation of induced pluripotent stem cells (iPSCs) [14] . However, it is not yet known whether the pluripotency-inducing and -maintaining activity of this gene pair is specific to mammals or existed in a more primitive vertebrate ancestor. Here we identify and isolate an axolotl Pou2 ( AxPou2 ) ortholog from a new contig assembly of ESTs. This finding provides the first evidence that a non-mammalian vertebrate has both the Pou2 and Oct4 genes, supporting the hypothesis that Oct4 emerged at least as early as the base of the tetrapod lineage [4] . Second, we show that AxPou2 , axolotl Oct4 ( AxOct4 ), xenopus Oct91 , as well as medaka Pou2 are each able to act together with mouse Sox2 , Klf4 and Myc to generate pluripotent cells from mouse fibroblasts, indicating that Oct4 as well as Pou2 homologues have pluripotency-inducing activities. These results also show that the previously observed inability of zebrafish Pou2 to sustain a pluripotent cell state is a property specific to this species and is not representative of all teleost Pou2 genes. Finally, we show that AxOct4 and AxPou2 can induce a pluripotent cell state in human fibroblasts and generate iPSCs. On the basis of these results, we conclude that the activity to support pluripotency is an ancient feature of the vertebrate Pou2 and Oct4 genes that existed before the emergence of the Oct4 gene—a process that occurred at least at the base of the tetrapod lineage. AxPou2 identification, synteny and phylogenesis To determine whether a Pou2 ortholog distinct from the existing putative Oct4 sequence [6] could be identified in axolotl, we performed a BLAST search on a contig assembly of ESTs derived from Sanger and 454 sequences using the AxOct4 sequence, and found a single partial sequence that was similar but distinct from Oct4 . BLAST searching of the RefSeq database with this new sequence showed that its closest orthologs were vertebrate Pou2 family members. Finally, a long-insert cDNA library was screened to obtain the full coding sequence. These results indicate that the axolotl harbours two distinct genes encoding for class V Pou domain proteins. To assign gene orthology to the putative AxPou2 and the previously identified AxOct4 sequences, phylogenetic analysis of Pou2 and Oct4 homologue sequences from different species was performed based on a multiple sequence alignment of the DNA-binding domains ( Supplementary Fig. S1 ). The analysis resulted in two main branches where Oct4 and Pou2 gene sequences segregated. The phylogenetic tree assigned the new AxPou2 sequence in a cluster with the chicken, opossum, tammar and platypus Pou2 sequences ( Fig. 1a ). The medaka, stickleback, cod, carp and zebrafish Pou genes clustered in a separate Pou2 subbranch, whereas the xenopus POU orthologs formed a distinct cluster consistent with an independent duplication event of the POU class V ancestor gene in this organism. In contrast, AxOct4 formed a cluster together with the Oct4 sequences from lizard, platypus, tammar and eutherian mammals ( Fig. 1a ). These results indicate that axolotl—similar to marsupials and monotremes—harbours bona fide Pou2 and Oct4 orthologs and that Pou2 / Oct4 ortholog genes can be traced back to a gene duplication event at the base of the tetrapod lineage. 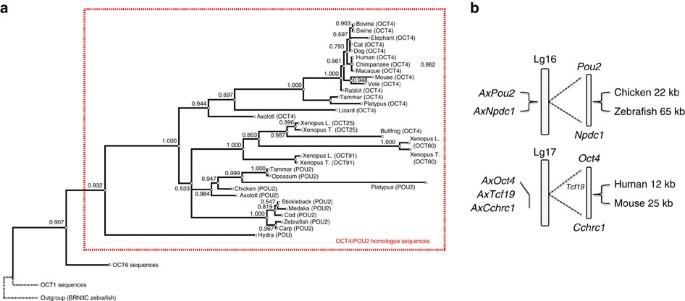Figure 1: Phylogenetic and syntenic analysis ofAxOct4andAxPou2. (a) Phylogenetic tree of the Oct4 and Pou2 homologues from different species based on the alignment of the POU sequences indicates that axolotl has both thePou2andOct4homologues. The branches are shown with their calculated relative lengths and the posterior probabilities are labelled at the corresponding nodes. The outgroup (BRN3C), the Oct1 and Oct6 sequences and the dotted branches are shown to emphasize the split of the subtree of theOct4/Pou2sequences. The length of the dotted branches is arbitrary. SeeSupplementary Fig. S1for sequence alignment. (b) Assignment ofAxPou2andAxOct4toAmbystomalinkage group 16 and 17, respectively.AxPou2mapped to the position ofAxNpdc1(20 cM) andAxOct4(76 cM) mapped to the position ofAxTcf19andAxCchrc1. ThePou2-Npdc1andOct4-TCf19-Cchcr1linkage relationships are observed as conserved syntenies in chicken–zebrafish and mouse–human, respectively. Figure 1: Phylogenetic and syntenic analysis of AxOct4 and AxPou2 . ( a ) Phylogenetic tree of the Oct4 and Pou2 homologues from different species based on the alignment of the POU sequences indicates that axolotl has both the Pou2 and Oct4 homologues. The branches are shown with their calculated relative lengths and the posterior probabilities are labelled at the corresponding nodes. The outgroup (BRN3C), the Oct1 and Oct6 sequences and the dotted branches are shown to emphasize the split of the subtree of the Oct4 / Pou2 sequences. The length of the dotted branches is arbitrary. See Supplementary Fig. S1 for sequence alignment. ( b ) Assignment of AxPou2 and AxOct4 to Ambystoma linkage group 16 and 17, respectively. AxPou2 mapped to the position of AxNpdc1 (20 cM) and AxOct4 (76 cM) mapped to the position of AxTcf19 and AxCchrc1 . The Pou2-Npdc1 and Oct4-TCf19-Cchcr1 linkage relationships are observed as conserved syntenies in chicken–zebrafish and mouse–human, respectively. Full size image To verify the orthologous relationship between AxOct4 and AxPou2 with Oct4 and Pou2 genes, respectively, a study on conserved synteny was performed. To this end, the positions of AxPou2 and AxOct4 within the axolotl genetic linkage map were determined using the AxTg mapping panel [15] . AxPou2 mapped to the position of AxNpdc1 (LG16, 20 cM) and AxOct4 mapped to the position of AxCchcr1 and AxTcf19 (LG17, 76 cM). Tight physical linkage of Pou2-Npdc1 was observed in chicken and zebrafish, and tight physical linkage of Oct4-Cchcr1-Tcf19 was observed in human and mouse ( Fig. 1b ). Therefore, these results establish the orthology of Ax Pou2 to Pou2 , and AxOct4 to Oct4 . Next, we examined the localization of AxPou2 by in situ hybridization. Similar to AxOct4 (ref. 6 ), AxPou2 was expressed in the surface ectoderm of stage-11 embryos, which would be equivalent to the epiblast stage in mammals ( Fig. 2a ). By stage 20, similar to the zebrafish Pou2 , expression was observed in the brain ( Fig. 2a ). This expression data supports the notion that AxPou2 is a bona fide Pou2 and not an Oct4 family member. In addition, AxPou2 expression was observed in gonia of 3 cm-long larvae. The expression pattern overlapped with that of axolotl c-kit, which had previously been reported to be expressed in gonia [6] ( Fig. 2b ). Interestingly, we also observed expression of AxOct4 in the gonads ( Fig. 2b ). In summary, our data indicates that the axolotl, a representative of caudate amphibia, has both Pou2 and Oct4 homologues, similar to marsupial and monotreme mammals, supporting the previous hypothesis that Oct4 arose at least as early as the base of the tetrapod lineage. 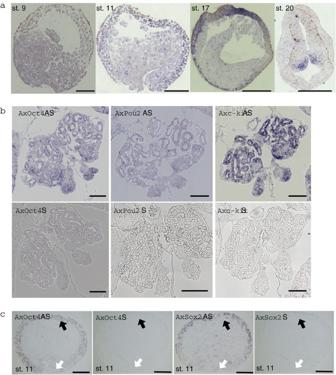Figure 2: Localization ofAxOct4,AxPou2andAxSox2in axolotl embryos. (a) Expression ofAxPou2mRNA during embryonic development of axolotl.AxPou2showed a weak expression signal in stage-9 blastula-stage embryos.AxPou2was expressed in the ectoderm of animal cap and blastopore lip of a stage-11 (early gastrulation) embryo and in the ectoderm of stage-17 neurula-stage embryos. At stage 20, a large signal is seen in the neural tube in the hindbrain region (right) during neurulation and in the hindbrain in somite-stage embryos.In situhybridization was performed on paraffin section (10-μm thick). Image was taken in bright field (NA 0.8); scale bar, 500 μm. st, stage. (b)AxOct4,AxPou2andAxc-kitmRNA are present in gonia during development of axolotl. Sense control probes show no background signal. The negative control using the sense probe is indicated with S, and the specific signal from the antisense probe is labelled with AS.In situhybridization was performed on paraffin section (10 μm thick) of 3-cm axolotl larvae. Image was taken in bright field (NA 0.8); scale bar, 100 μm. (c)AxOct4andAxSox2RNAin situhybridization in a stage-11 axolotl embryo (38.5 h post fertilization). The negative control using the sense probe is indicated with S, and the specific signal from the antisense probe is labelled with AS. The black arrows mark the axolotl animal cap (equivalent to the mouse epiblast); the white arrows mark the axolotl blastopore lip (equivalent to the mouse primitive streak). Scale bars, 500 μm. Figure 2: Localization of AxOct4 , AxPou2 and AxSox2 in axolotl embryos. ( a ) Expression of AxPou2 mRNA during embryonic development of axolotl. AxPou2 showed a weak expression signal in stage-9 blastula-stage embryos. AxPou2 was expressed in the ectoderm of animal cap and blastopore lip of a stage-11 (early gastrulation) embryo and in the ectoderm of stage-17 neurula-stage embryos. At stage 20, a large signal is seen in the neural tube in the hindbrain region (right) during neurulation and in the hindbrain in somite-stage embryos. In situ hybridization was performed on paraffin section (10-μm thick). Image was taken in bright field (NA 0.8); scale bar, 500 μm. st, stage. ( b ) AxOct4 , AxPou2 and Axc-kit mRNA are present in gonia during development of axolotl. Sense control probes show no background signal. The negative control using the sense probe is indicated with S, and the specific signal from the antisense probe is labelled with AS. In situ hybridization was performed on paraffin section (10 μm thick) of 3-cm axolotl larvae. Image was taken in bright field (NA 0.8); scale bar, 100 μm. ( c ) AxOct4 and AxSox2 RNA in situ hybridization in a stage-11 axolotl embryo (38.5 h post fertilization). The negative control using the sense probe is indicated with S, and the specific signal from the antisense probe is labelled with AS. The black arrows mark the axolotl animal cap (equivalent to the mouse epiblast); the white arrows mark the axolotl blastopore lip (equivalent to the mouse primitive streak). Scale bars, 500 μm. Full size image Reprogramming to pluripotency is an ability of Pou2 homologues To further delve into the functional relationships of the POU orthologs, we surveyed the relative activity of the human OCT4, mouse Oct4, xenopus Oct91, AxPou2, AxOct4, medaka Pou2 and zebrafish Pou2 to support the formation of iPSCs in reprogramming assays. Mouse embryonic fibroblasts (MEFs) that contained a green fluorescent protein (GFP) transgene driven by the mouse Oct4 promoter [16] were transduced with retroviruses encoding mouse Sox2 , mouse Klf4 and mouse c-Myc , plus one of each different POU homologues. The reprogramming efficiency corresponds to the percentage of cells that were able to reactivate GFP expression 14 days after transduction ( Fig. 3a ). Among the non-mammalian POU factors, xenopus Oct91 was almost as efficient as the mouse and human Oct4 cDNAs in generating GFP+ cells. In contrast, medaka Pou2 , AxPou2 and AxOct4 exhibited a lower reprogramming efficiency. Finally, iPSC colonies could not be established when using zebrafish Pou2 , which is consistent with the inability of zebrafish Pou2 to sustain a pluripotent cell state in mouse ESCs [9] . Three different iPSC colonies were picked for each homologue and genotyped to exclude cross-contamination among the different POU factors ( Supplementary Fig. S2 ). The iPSC lines were labelled as H, M, X, AP, A and K, corresponding to human OCT4 , mouse Oct4 , xenopus Oct91 , AxPou2 , AxOct4 and medaka Pou2 , respectively, and followed by a number that distinguishes the different clonal cell lines established from each homologue. All colonies were able to reactivate and maintain the expression of the Oct4 -GFP transgene and stained positive for alkaline phosphatase (ALP) ( Fig. 3b and Supplementary Fig. S3 ). In addition, the expression of the mouse pluripotent markers Oct4 , Nanog , Fgf4 , Utf1 and Rex1 was analysed by quantitative RT–PCR (qRT–PCR) ( Fig. 3c ). All clones exhibited levels of expression similar to those of two different mouse ESC lines used as a positive control, and different from that of the initial fibroblastic population, thus, demonstrating successful reprogramming. Finally, a teratoma assay was performed to assess the in vivo pluripotency capacity. As expected, all clones were able to differentiate into all three germ layers ( Fig. 4 ). In summary, all POU homologues, except for zebrafish, were able to stably induce pluripotency in mouse fibroblasts and generate bona fide iPSCs. These results indicate that the inability of the zebrafish Pou2 to support pluripotency is not representative of all teleost Pou2 genes. Indeed, the medaka and axolotlPou2 orthologs were at least as potent as AxOct4 in our reprogramming assays. This data indicate that the ability to reprogram cells to a pluripotent-like state is an ancient trait of Pou2 and Oct4 homologues. 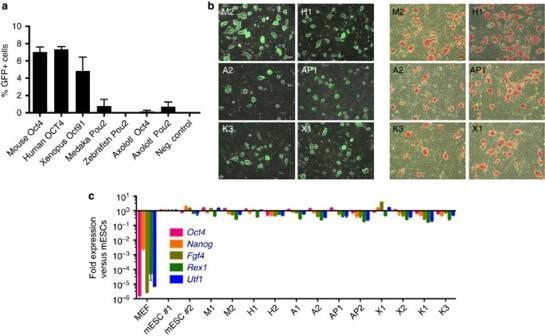Figure 3: Generation and characterization of mouse iPSCs generated using differentPOUfactors. (a) MEFs containing a GFP transgene driven by theOct4promoter were transduced with pMX retroviruses coding for mouseSox2, mouseKlf4, mousec-Mycand one of each of thePOUhomologues. After 14 days of transduction, the number of GFP-positive cells was measured by fluorescence-activated cell sorting and plotted as a percentage of the total number of cells, thus indicating the reprogramming efficiency. s.d. corresponds to two independent experiments that were run in parallel. (b) For eachPOUfactor, one iPSC clonal cell line is shown for GFP and ALP expression. (c) Expression of endogenous pluripotency markers was measured by qRT–PCR in two clonal iPSC cell lines established using each differentPOUfactor, MEFs and in two mESC cell lines. All data are calibrated to mESCs #1, which is considered to be 1. Error bars reflect the s.e.m. based on technical replicates. A,AxOct4; AP,AxPou2, X, XenopusOct91; K, MedakaPou2; H, HumanOCT4; M, MouseOct4. Scale bars, 100 μm. Figure 3: Generation and characterization of mouse iPSCs generated using different POU factors. ( a ) MEFs containing a GFP transgene driven by the Oct4 promoter were transduced with pMX retroviruses coding for mouse Sox2 , mouse Klf4 , mouse c-Myc and one of each of the POU homologues. After 14 days of transduction, the number of GFP-positive cells was measured by fluorescence-activated cell sorting and plotted as a percentage of the total number of cells, thus indicating the reprogramming efficiency. s.d. corresponds to two independent experiments that were run in parallel. ( b ) For each POU factor, one iPSC clonal cell line is shown for GFP and ALP expression. ( c ) Expression of endogenous pluripotency markers was measured by qRT–PCR in two clonal iPSC cell lines established using each different POU factor, MEFs and in two mESC cell lines. All data are calibrated to mESCs #1, which is considered to be 1. Error bars reflect the s.e.m. based on technical replicates. A, AxOct4 ; AP, AxPou2 , X, Xenopus Oct91 ; K, Medaka Pou2 ; H, Human OCT4 ; M, Mouse Oct4 . Scale bars, 100 μm. 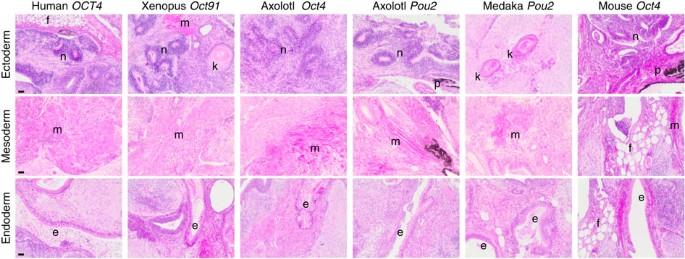Figure 4: Teratoma assay of mouse iPSCs generated using differentPOUfactors. Hematoxylin and eosin-stained sections of teratomas formed 4 weeks after subcutaneously injecting nude mice with mouse iPSCs generated using the different POU factors. Teratomas contain all three embryonic germ layers: endoderm (respiratory epithelium (e)), mesoderm (cartilage (c), skeletal muscle (m), adipose tissue (f)) and ectoderm (neural epithelium with rosettes (n), pigmented melanocytes (p)). Scale bars, 100 μm. Full size image Figure 4: Teratoma assay of mouse iPSCs generated using different POU factors. Hematoxylin and eosin-stained sections of teratomas formed 4 weeks after subcutaneously injecting nude mice with mouse iPSCs generated using the different POU factors. Teratomas contain all three embryonic germ layers: endoderm (respiratory epithelium (e)), mesoderm (cartilage (c), skeletal muscle (m), adipose tissue (f)) and ectoderm (neural epithelium with rosettes (n), pigmented melanocytes (p)). Scale bars, 100 μm. Full size image Axolotl Oct4 , Pou2 and Sox2 can reprogram human cells Axolotl is the most basal tetrapod containing both an Oct4 and Pou2 homologue. In addition, the AxOct4 gene appears to be the most ancient Oct4 ortholog identified to date. For these reasons, we sought to further characterize the reprogramming ability of AxOct4 and AxPou2 in human fibroblasts, a rather advanced species in evolution. In human and mouse ESCs, Oct4 protein interacts with Sox2 to activate downstream genes that maintain the pluripotency network, and both factors are essential for the generation of iPSCs [17] . We therefore assessed the efficiency of generation of human iPSCs (hiPSCs) when AxOct4 and AxPou2 were used in combination with either human or axolotl Sox2 (AxSox2). As early embryonic expression of AxSox2 has not been previously described, we first confirmed that AxSox2 was co-expressed with AxOct4 in the ectoderm of stage-11 embryos ( Fig. 2c ). To generate hiPSCs, retroviruses encoding human OCT4 (O), SOX2 (S), KLF4 (K), c-MYC (M), as well as AxOct4 (o), AxPou2 (a) and AxSox2 (s) were used to transduce two primary human fibroblast cell lines: hFib1 and hFib2 ( Fig. 5a ). hiPSC lines derived from hFib1 and hFib2 cells, which were termed iPS1 and iPS2, respectively, were established from all the tested combinations, with the image of a representative colony shown in Fig. 5a . All colonies were genotyped by PCR to confirm the presence of only the expected transgenes ( Supplementary Fig. S4 ). The reprogramming efficiency of the combinations is indicated in Supplementary Table S1 . The hESC cell line H9 and an iPSC cell line generated only with human factors were used as positive controls ( Fig. 5a ). 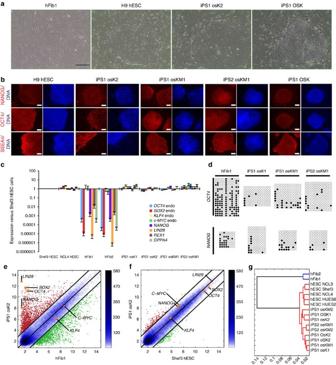Figure 5: Generation and characterization of hiPSCs generated usingAxolotl Oct4andAxSox2. (a) Representative images showing an iPSC colony generated using the axolotl factors in comparison with the initial hFib1 population, as a negative control, and iPSCs generated with only human factors (OSK) and H9 hESCs, as positive controls. Scale bars, 500 μm. (b) Immunofluorescence analysis of NANOG, OCT4 and SSEA4 on iPS1 osK2, iPS1 osKM1 and iPS2 osKM1 cell lines. Human ESC line H9 and OSK iPSC cell line were used as positive controls. Nuclei were stained with Hoechst (blue). Scale bars, 500 μm. (c) Expression of endogenous pluripotency markers in hFib1, hFib2, iPS1 osK1, iPS1 osK2, iPS1 osKM1 and iPS2 osKM1 cell lines as well as in Shef3 and NCL4 hESCs was measured by qRT–PCR and plotted relative to Shef3 hESC levels. Error bars reflect s.e. based on normalization toGAPDHandACTB(housekeeping genes). (d) Bisulfite sequencing of genomicOCT4andNANOGpromoter regions. Open and closed circles indicate unmethylated and methylated CpGs, respectively. (e–g) Pairwise scatter plots of global gene expression profiles comparing iPS1 osK2 cells with human hFib1 cells (e) and Shef3 hESCs (f). Black lines indicate a two-fold change in gene expression levels between the paired populations. Colour bar on the right indicates scattering density. Genes up- and downregulated are shown by red and green circles, respectively. The position of the pluripotency marker genesOCT4,SOX2,NANOG,KLF4,LIN28andc-MYCis represented as orange circles. (g) Hierarchical clustering, with blue branches connecting human fibroblasts and red branches connecting pluripotent cell populations (iPSCs or hESCs). Figure 5: Generation and characterization of hiPSCs generated using Axolotl Oct4 and AxSox2 . ( a ) Representative images showing an iPSC colony generated using the axolotl factors in comparison with the initial hFib1 population, as a negative control, and iPSCs generated with only human factors (OSK) and H9 hESCs, as positive controls. Scale bars, 500 μm. ( b ) Immunofluorescence analysis of NANOG, OCT4 and SSEA4 on iPS1 osK2, iPS1 osKM1 and iPS2 osKM1 cell lines. Human ESC line H9 and OSK iPSC cell line were used as positive controls. Nuclei were stained with Hoechst (blue). Scale bars, 500 μm. ( c ) Expression of endogenous pluripotency markers in hFib1, hFib2, iPS1 osK1, iPS1 osK2, iPS1 osKM1 and iPS2 osKM1 cell lines as well as in Shef3 and NCL4 hESCs was measured by qRT–PCR and plotted relative to Shef3 hESC levels. Error bars reflect s.e. based on normalization to GAPDH and ACTB (housekeeping genes). ( d ) Bisulfite sequencing of genomic OCT4 and NANOG promoter regions. Open and closed circles indicate unmethylated and methylated CpGs, respectively. ( e – g ) Pairwise scatter plots of global gene expression profiles comparing iPS1 osK2 cells with human hFib1 cells ( e ) and Shef3 hESCs ( f ). Black lines indicate a two-fold change in gene expression levels between the paired populations. Colour bar on the right indicates scattering density. Genes up- and downregulated are shown by red and green circles, respectively. The position of the pluripotency marker genes OCT4 , SOX2 , NANOG , KLF4 , LIN28 and c-MYC is represented as orange circles. ( g ) Hierarchical clustering, with blue branches connecting human fibroblasts and red branches connecting pluripotent cell populations (iPSCs or hESCs). Full size image Next, we sought to characterize the molecular properties of the generated hiPSC lines. To this end, we first assessed the expression of several pluripotency markers by immunochemistry. The generated iPSCs stained negative for the non-pluripotency marker stage-specific embryonic antigen 1 (SSEA-1) ( Supplementary Fig. S5 ) and positive for the pluripotency markers OCT4, NANOG, SSEA4, TRA1-60 and TRA1-81, exhibiting levels similar to those in H9 hESCs ( Figs 5b and 6a and Supplementary Fig. S5 ). Second, the mRNA levels of the endogenous pluripotency markers OCT4 , SOX2 , KLF4 , c-MYC , NANOG , REX1 , LIN28 and DPPA4 as determined by qRT–PCR were comparable to those in Shef3 and NCL4 hESC lines ( Figs 5c and 6b and Supplementary Fig. S6 ). Next, bisulfite sequencing analysis of the OCT4 and NANOG promoter regions showed that both promoters became demethylated during the reprogramming process ( Fig. 5d ). In addition, the retroviral transgenes were silenced, as revealed by qRT–PCR ( Fig. 6c and Supplementary Fig. S6 ). Finally, the global gene expression profiles of several iPSC lines were compared with those of human fibroblasts and hESCs by microarray analysis. Pairwise scatter plot comparison of the iPS1 osK2 cell line with the parental hFib1 cells ( Fig. 5e ) and Shef3 hESCs ( Fig. 5f ) showed that iPS1 osK2 cells exhibited a fully reprogrammed gene expression profile, similar to that of Shef3 hESCs but completely different from that of hFib1 cells. As expected, all iPSC lines showed a similar gene expression profile ( Supplementary Fig. S6 ). Finally, the generated iPSCs clustered close together with hESCs but not with the parental hFib cells, as seen in a hierarchical analysis ( Fig. 5g ). In summary, our results indicate that AxOct4 and AxPou2 could reprogram the human fibroblastic transcriptional network into a de novo pluripotent cell state. 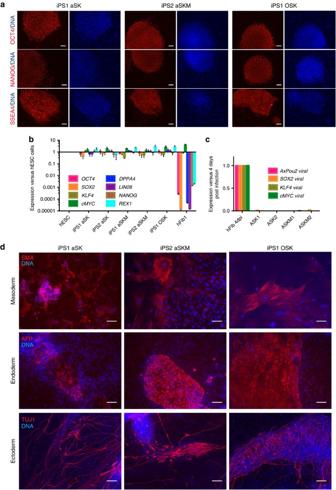Figure 6: Characterization of hiPSCs generated usingAxPou2. (a) Immunofluorescence analysis of NANOG, OCT4 and SSEA4 on iPS1 aSK and iPS2 aSKM cell lines. OSK iPSC cell line was used as a positive control. Nuclei were stained with Hoechst (blue). Scale bars, 500 μm. (b) Expression of endogenous pluripotency markers in hFib1, iPS1 aSK, iPS1 aSKM, iPS2 aSK and iPS2 aSKM cell lines as well as in Shef3 hESCs was measured by qRT–PCR and plotted relative to Shef3 hESC levels. Error bars reflect s.e. based on normalization toGAPDHandACTB(housekeeping genes). (c) Expression level of the viral transgenes in hiPSCs was measured by qRT–PCR using specific primers. Fibroblasts collected 4 days after infection are used for comparison as a positive control. Error bars represent the s.e. arising from usingGAPDHandACTBfor normalization. (d)In vitrodifferentiation of the AxPou2 hiPSCs into cells of all three germ layers as shown by immunocytochemistry: endoderm (α-fetoprotein, AFP), mesoderm (α-smooth muscle actin, SMA), and ectoderm (β-Tubulin IIIb, TUJ1). Nuclei were stained with Hoechst (blue). Scale bars, 250 μm. Figure 6: Characterization of hiPSCs generated using AxPou2 . ( a ) Immunofluorescence analysis of NANOG, OCT4 and SSEA4 on iPS1 aSK and iPS2 aSKM cell lines. OSK iPSC cell line was used as a positive control. Nuclei were stained with Hoechst (blue). Scale bars, 500 μm. ( b ) Expression of endogenous pluripotency markers in hFib1, iPS1 aSK, iPS1 aSKM, iPS2 aSK and iPS2 aSKM cell lines as well as in Shef3 hESCs was measured by qRT–PCR and plotted relative to Shef3 hESC levels. Error bars reflect s.e. based on normalization to GAPDH and ACTB (housekeeping genes). ( c ) Expression level of the viral transgenes in hiPSCs was measured by qRT–PCR using specific primers. Fibroblasts collected 4 days after infection are used for comparison as a positive control. Error bars represent the s.e. arising from using GAPDH and ACTB for normalization. ( d ) In vitro differentiation of the AxPou2 hiPSCs into cells of all three germ layers as shown by immunocytochemistry: endoderm (α-fetoprotein, AFP), mesoderm (α-smooth muscle actin, SMA), and ectoderm (β-Tubulin IIIb, TUJ1). Nuclei were stained with Hoechst (blue). Scale bars, 250 μm. Full size image HiPSC lines generated using axolotl factors are pluripotent Next, we assessed the pluripotent potential of the generated iPSC lines. The differentiation potential of iPSCs in vitro was investigated by embryoid body (EB) formation. EBs were generated by the hanging-drop method and cells were induced to differentiate. After 2 weeks of differentiation, specific cell types of all three germ layers were observed—that is, cells stained positive for the endoderm marker alpha-fetoprotein, the mesoderm marker α-smooth muscle actin and the ectoderm marker β-Tubulin IIIb, as detected by immunofluorescence microscopy ( Figs 6d and 7a and Supplementary Fig. S7 ). The in vivo differentiation potential of iPSCs generated using AxOct4 was additionally evaluated by teratoma formation. After 6–8 weeks of subcutaneous injection of iPSC lines into nude athymic mice, teratomas containing tissues of all three germ layers had formed from all lines analysed ( Fig. 7b and Supplementary Fig. S7 ). The teratoma assay is the gold standard for assessing the pluripotency of human ESCs. However, more stringent methods can be used to evaluate pluripotency using the mouse model. Mouse iPSCs generated using AxOct4 ( Fig. 3 ) were thus aggregated with mouse morula-stage embryos ( Supplementary Fig. S8 ) and shown to generate chimeric mice ( Supplementary Fig. S8 ), demonstrating the ability of AxOct4 to induce bona fide pluripotency. Germline contribution was observed by the presence of GFP+ cells in the gonads of 13.5-days post-coitum (d.p.c.) female embryos ( Supplementary Fig. S8 ). Taken together, these data indicate that iPSC lines can be generated from fibroblasts of two different mammalian species using the AxOct4 and AxPou2 genes, and that these iPSC lines exhibit the pluripent capacity to differentiate into cells of all three germ layers. 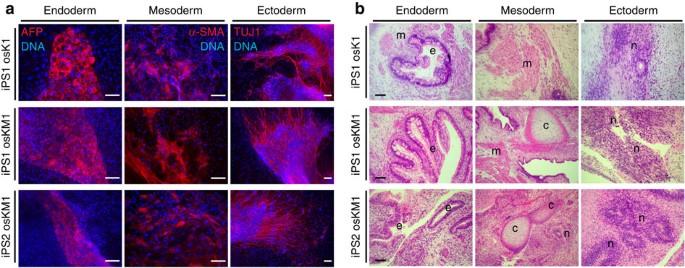Figure 7:In vivoandin vitrodifferentiation of iPSCs generated usingAxOct4andAxSox2. (a)In vitrodifferentiation into cells of all three germ layers as shown by immunocytochemistry: endoderm (α-fetoprotein, AFP), mesoderm (α-smooth muscle actin, SMA) and ectoderm (β-Tubulin IIIb, TUJ1). Nuclei were stained with Hoechst (blue). Scale bars, 250 μm. (b) Microsections of hematoxylin and eosin-stained teratoma formed within 6–8 weeks of injecting nude mice with iPSCs generated using axolotl factors plus human factors. iPSCs had differentiated into tissues of all three germ layers: endoderm (respiratory epithelium (e)), mesoderm (cartilage (c), skeletal muscle (m)), and ectoderm (neural epithelium with rosettes (n)). Scale bars, 100 μm. Figure 7: In vivo and in vitro differentiation of iPSCs generated using AxOct4 and AxSox2 . ( a ) In vitro differentiation into cells of all three germ layers as shown by immunocytochemistry: endoderm (α-fetoprotein, AFP), mesoderm (α-smooth muscle actin, SMA) and ectoderm (β-Tubulin IIIb, TUJ1). Nuclei were stained with Hoechst (blue). Scale bars, 250 μm. ( b ) Microsections of hematoxylin and eosin-stained teratoma formed within 6–8 weeks of injecting nude mice with iPSCs generated using axolotl factors plus human factors. iPSCs had differentiated into tissues of all three germ layers: endoderm (respiratory epithelium (e)), mesoderm (cartilage (c), skeletal muscle (m)), and ectoderm (neural epithelium with rosettes (n)). Scale bars, 100 μm. Full size image The evolution of the Oct4 gene and the origin of its pluripotency-supporting properties has been the subject of controversy [4] , [5] . Our data indicate that the axolotl has retained both the Pou2 and Oct4 genes, a property seen previously only in marsupials and monotremes [4] , [5] . The consensus trees ( Fig. 1a ) showed a clear separation of the Pou2 and Oct4 homologue sequences, indicating a possible gene duplication event that took place at least at the base of the tetrapod lineage, as previously suggested [4] . Interestingly, the recently identified Pou domain gene from hydra [18] appears to have the features of an Oct4 / Pou2 precursor gene, as shown in Fig. 1a , suggesting that the common Oct4 / Pou2 ancestor could have already existed even before the specification of vertebrates. We show that both AxPou2 and AxOct4 can reprogram mouse and human fibroblasts to a pluripotent cell state. Therefore, our data strongly indicate that the ancestral Oct4/Pou2 gene had the ability to induce and support pluripotency. A previous study found that although both the Oct4 and Pou2 genes are expressed in pluripotent tissues of the marsupial tammar, only Oct4 is expressed in the germ cell lineage [4] . AxOct4 could not previously be detected in axolotl germ cells [6] ; our data however indicate that AxOct4 and AxPou2 are both expressed in pluripotent tissues and germ cells. Thus, axolotl is the first species described to contain both Oct4 and Pou2 genes and to have both homologues expressed in its germ cells. Further experiments are required to determine whether AxPou2 is sufficient to maintain the germ cell fate in the absence of its Oct4 homologue. As with AxPou2 expression, medaka Pou2 expression is detected in germ cells but its function is still unclear [19] . However, as medaka does not contain an Oct4 homologue, it is reasonable to speculate that medaka Pou2 has a role in germ cell development. Taken together, these observations imply that the ancestral Oct4 / Pou2 gene could have had a role not only in pluripotency, but also in germ cell development—an ability that was selectively lost in some species during evolution. Tammar Oct4 is able to sustain pluripotency in mouse Oct4- null ESCs much more efficiently than tammar Pou2 . These observations were reproduced using Oct4 and Pou2 homologues from different species, suggesting that Pou2 factors have a reduced ability to maintain pluripotency compared with Oct4 factors. In our reprogramming experiments, we generated iPSC colonies from medaka Pou2 and AxPou2 . In fact, using AxPou2 we generated more iPSC colonies than using AxOct4 . These results indicate that the ancestral Oct4 / Pou2 gene exhibited a full pluripotent potential that was maintained after Oct4 arose. However, after a certain point in evolution, Pou2 appears to have progressively lost part of its pluripotent potential while maintaining or acquiring new somatic functions. Although we detected some GFP-positive cells using zebrafish Pou2 , we could not establish any iPSC colonies. In agreement with this result, the zebrafish Pou2 gene does not support mouse ESC pluripotency in the absence of mouse Oct4 (refs. 5 , 9 ). Our results indicate that the limited potential of zebrafish Pou2 to induce and maintain pluripotency is specific to zebrafish, and does not apply to all Pou2 orthologs, as axolotl and medaka Pou2 were able to generate iPSC colonies. Transcription factors modulate transcription by binding to DNA target sequences and recruiting components of the transcription machinery by their transactivation domains [20] . To investigate the inability of zebrafish Pou2 to induce pluripotency, we assessed its DNA binding and transactivation activity ( Supplementary Fig. S9 ) in comparison with other POU homologues. The zebrafish POU2 protein showed a transactivation activity level comparable to those of other POU factors in a luciferase assay ( Supplementary Fig. S9 ). Thus, the inability of the zebrafish POU factor to induce pluripotency was not due to a lack of DNA-binding or transactivation activity. As mentioned previously, heterodimer formation between OCT4 and SOX2 via the POU domain and HMG domain, respectively, is essential for pluripotency [21] . To exclude that the inability of the zebrafish ortholog to generate iPSCs was due to an absence of interaction with mouse Sox2, we generated models to evaluate in silico the electrostatic interactions between the HMG domain and the POU domain of each homologue ( Supplementary data and Supplementary Fig. S9 ). Our analysis revealed that the interaction between the HMG domain of SOX2 and the region between the α 3 helix and the α 1 –α 2 loop of the POU HD domain is highly conserved among all homologues. In comparison, the interacting region with SOX2 on the HOXB1-like DNA promoters is less conserved. This suggests that the interaction of POU homologues with mouse SOX2 could be partially altered on certain promoters, which could also explain the lower reprogramming efficiency. However, this is mere speculation, as the importance of different recognition motifs for successful reprogramming has not yet been determined. In this study, we focused on the highly conserved POU domain, but it is likely that further crucial properties are encrypted in the transactivation domains, which have not yet been extensively studied. In summary, our analysis could not explain the inability of the zebrafish POU2 protein to induce pluripotency. Thus, future investigations should unveil all the properties of POU factors required for successful reprogramming. Finally, with this study, we are the first group to show a pluripotency-related role for AxSox2. AxPou2, AxOct4 and/or AxSox2, in combination with the other three/two human factors, could induce pluripotent cell formation in human fibroblasts, indicating that AxPou2, AxOct4 and AxSox2 cannot only substitute for the human homologues, but also effectively dimerize with the human proteins. Our results indicate that the Oct4 and Sox2 pluripotency-inducing activity is conserved between axolotl and human, and suggest that the two transcription factors are components of the pluripotency circuitry conserved among vertebrates. Although intraspecies reprogramming has already been described [22] , [23] , to our knowledge this is the first study reporting the successful reprogramming of human somatic cells with Oct4 and Sox2 transcription factors from lower vertebrates. Our results, together with the previously reported work on axolotl Nanog [24] , [25] , encourage the derivation of pluripotent stem cells from axolotl, wherein the key factors in the pluripotency network are present and functional. Oct4, Pou2 and Sox2 ortholog amplification and cloning A contig assembly of axolotl sequences derived from Sanger [26] , [27] , 454 (ref. 28 ), and unpublished 454 sequences were assembled using MIRA 3.0. The AxPou2 sequence was identified by querying the contig assembly with the AxOct4 sequence via BLAST. A sequence fragment was identified, which when BLASTed to NCBI RefSeq set, identified Pou2 sequences from different organisms as the closest ortholog. Full-length AxPou2 was identified by PCR from a long-insert cDNA library using primers designed from the identified contig sequence. The full-length gene was amplified by PCR (Axolotl-Pou2fl- Bam HI-Fw, Axolotl-Pou2- Not I-Rv) and directionally cloned into the pMXs vector using Bam HI and Not I restriction sites by standard methods. The vector pME18S-FL3 containing zebrafish Pou2 (ImaGenes) was used to amplify zebrafish Pou2 as two fragments (Zebrafish- Eco RI-Fw and Zebrafish-T-A-Rv, Zebrafish-T-A-Fw and Zebrafish- Xho I-Rv). The PCR fragments were purified (QIAGEN) and used as template for a third PCR reaction using Zebrafish- Eco RI-Fw and Zebrafish- Xho I-Rv primers. The PCR product was purified, the Pou2 sequence was excised using Eco RI and Xho I, and was then ligated into the same sites within the vector pMXs. The xenopus Oct91 gene in the vector pCS2 was a kind gift from the Knöchel lab (University of Ulm). The Oct91 sequence was amplified (Xenopus- Bam HI-Pou91-Fw, Xenopus- Xho I-Pou91-Rv), the PCR product purified and Oct91 excised using BamHI and XhoI , and ligated into the same sites within pMXs. The medaka Oct4 gene was amplified as two fragments (Medaka-Oct4- Hin dIII-Fw and Medaka-Oct4-NCBI-Rv, Medaka-Oct4-NCBI-Fw and Medaka-Oct4- Xho I-Rv). PCR fragments were purified and used as template for a third PCR reaction using Medaka-Oct4- Hin dIII-Fw and Medaka-Oct4- Xho I-Rv primers. Purified PCR product was digested using Hin dIII and Xho I and ligated into the same sites within pMXs. AxOct4 cDNA was PCR amplified from stage-11 embryonic cDNA using primers designed from a published sequence [6] Oct4 -RT-Fw3 and Oct4 -RT-Rv2. AxOct4 was digested using Bst XI and cloned into pMX. AxSox2 cDNA fragment was PCR amplified from day-6 tail blastema cDNA using Sox2 _D_Fw1 and Sox2 _D_Rv1 primers. 5′RACE and 3′RACE was carried out by using the Gene Racer Kit (Invitrogen) using primers Sox2 _sRv1 and Sox2 _sFw2, respectively. Full-length AxSox2 was amplified from day-6 tail blastema cDNA using Sox2 _full_Fw and Sox2 _full_Rv primers. Finally, AxSox2 was cloned into pMX using Bam HI and Xho I. The cloning primers are described in Supplementary Table S2 . Phylogenetic and synteny analysis The phylogenetic analysis was performed with MRBAYES 3.2 using Bayesian Inference to reconstruct consensus phylogenetic trees with the posterior probabilities estimated by Markov chain Monte Carlo methods [29] . We first created an alignment of Oct4, Pou2, Oct1 and Oct6 gene sequences across different species and the zebrafish Brn3c gene as an outgroup. We used Gblocks [30] to select the most suitable conserved block for the analysis, which was the DNA-binding domain. We performed the analysis using both the alignment of the entire sequence and that of the DNA-binding domain and observed no major differences between the two consensus trees. The only criteria for the outgroup was to be a single sequence from a different class of POU factors. We used the Jones model for amino-acid substitutions [31] with the rate heterogeneity modelled by a gamma distribution. Each consensus tree was calculated from two independent runs (four chains per run with one cold and three heated chains), of 500,000 tree generations each (samples taken every 1,000), after excluding 25% of samples. The convergence was measured by the s.d. of split frequencies, which was between 0.000 and 0.0677 for the tree presented in Fig. 1a . The sequences used for alignment and tree building are indicated in Supplementary Table S3 . Genetic linkage mapping was performed according to previous methods [15] . Primers were designed to amplify DNA fragments from AxPou2 and AxOct4 that contained diagnostic single-nucleotide polymorphisms that were informative for mapping using a primer extension genotyping method [32] . Markers were mapped using MultiPoint 2.2 (ref. 33 ) and the Kosambi [34] mapping function. Paraffin sections of axolotl embryos Axolotl embryos were staged [35] , dejellied and fixed for 4 h in MEM-FA (100 mM MOPS buffer, pH 7.4, 2 mM EGTA, 1 mM MgSO 4 , 1% or 3.7% formaldehyde) at room temperature, washed in PBS, dehydrated in an ethanol series, incubated in xylol (Roth), and embedded in paraffin (Roth). Cross-sections 10 μm thick were washed in xylol, rehydrated in an ethanol series and washed in PBS. Immunofluorescence staining on axolotl embryos Sections were treated with 200 mM glycine/0.3% Triton X-100 solution, followed by citrate pH 6 (Dako), and blocking in 10% goat serum for 1 h. Sections were incubated overnight with polyclonal rabbit anti- AxOct4 antibody (anti- AxOct4 was generated against amino acids 1–161 of Axolotl OCT4). Following PBS washes, sections were incubated with Alexa Fluor 555-labelled goat anti-rabbit IgG secondary antibody (Invitrogen) for 1 h. Nuclei were counterstained with Hoechst 33342. Digital images were taken on the Zeiss Observer Z1 microscope ( × 20 Plan-Apochromat, NA 0.8, Zeiss) with AxioCam MRm camera (Zeiss) and stitched using the AxioVision program. In situ hybridization on axolotl embryos In situ hybridization was performed at 70 °C using digoxigenin (Roche)-labelled Sox2 or Oct4 probe as described by Myat et al. [36] BMPlease provide the expansion for BM.Please provide the expansion for BM. purple (Roche) was applied for colorimetric detection, and sections were imaged in bright field (Olympus SZX12, DF PLAPO 1x PF). Cell culture Primary human skin fibroblasts were isolated from two Caucasian women—48-year-old (hFib1) and 33-year-old (hFib2)—and cultured for several passages in fibroblast medium, composed of DMEM high glucose, supplemented with 10% fetal bovine serum, 1% sodium pyruvate, 2 mM L-glutamine and penicillin/streptomycin (all PAA), on gelatin-coated culture dishes until infection. Human ESCs and iPSCs were cultured on mitomycin C–treated CF1 mouse feeder layers (Millipore) in human ESC medium, composed of Knockout DMEM, 20% Knockout serum replacement (Invitrogen), 1% nonessential amino acids, 0.10 mM β-mercaptoethanol (PAA), 2 mM L-glutamine and penicillin/streptomycin, supplemented with 5 ng ml −1 human basic fibroblast growth factor (Peprotech), and passaged as previously described [37] . MEFs were isolated from 13.5-d.p.c. OG2 embryos [16] and cultured in fibroblast medium as described above. Mouse ESCs and iPSCs were cultured on irradiated MEFs in mouse ESC medium, composed of Knockout DMEM (Invitrogen), 20% Knockout serum replacement (Invitrogen), 1% nonessential amino acids (PAA), 0.10 mM β-mercaptoethanol, 2 mM L -glutamine and penicillin/streptomycin, supplemented with leukemia inhibitory factor (LIF). Induction of pluripotent stem cells The moloney-based (pMXs) retroviral vectors with the cDNAs for human OCT4 , mouse Oct4 , xenopus Oct91 , zebrafish Pou2 , medaka Pou2 , AxOct4 , AxPou2 and AxSox2 as well as human and mouse SOX2 , KLF4 and c-MYC were cotransfected with packaging helper plasmids into 293T cells using Fugene 6 transfection reagent (Roche) [22] , [38] . Viral supernatants were collected 48 h later, filtered and used directly for infection. Human fibroblasts were plated on gelatin-coated six-well plates at a density of 50,000 cells per well 1 day before the first infection. Fibroblasts were incubated twice with viral supernatants containing combinations of equal amounts of each virus and supplemented with 6 μg ml −1 protamine sulphate (Sigma Aldrich) for 24 h. The day after the second infection, fibroblasts were reseeded at a density of 25,000 or 50,000 cells per well on gelatin-coated six-well plates in human fibroblast medium. One day later, the medium was switched to human ESC medium supplemented with 1 mM valproic acid (Sigma Aldrich). Valproic acid was withdrawn once human ESC-like colonies were visible. iPSC colonies were mechanically isolated within 3–7 weeks of infection and were replated and maintained on CF1 MEF feeder cells (Millipore) in human ESC medium. The AxOct4 hiPSC reprogramming experiment was repeated twice using two different fibroblast cell lines, hFib1 and hFib2, each time. The AxPou2 hiPSC reprogramming experiment was performed once using both hFib1 and hFib2, demonstrating its reproducibility. Mouse iPSCs using all different POU factors were generated as previously described [14] . Two independent experiments using duplicates for each Pou factor were performed. The percentage of mouse reprogrammed GFP-positive cells was measured using a FACSAria cell sorter (BD Bioscience) 14 days after infection. After sorting, GFP-positive cells were plated on irradiated MEFs from which single-cell colonies were picked and expanded. iPSC characterization ALP staining, immunohistochemistry, qRT–PCR, bisulfite sequencing, genotyping and in vivo teratoma formation were performed as previously described [39] , [40] , [41] . Clonal iPSC lines at passage 5 were characterized. In vitro differentiation of hiPSCs EBs were generated from hiPSCs using the hanging-drop method in MEF-conditioned medium, supplemented with Y27632 10 μM (Ascent Scientific), for 5 days (1,000 cells per 30 μl drop). EBs were plated on gelatin-coated plates and cultured for 14 days in different media. The following media were used to direct differentiation into specific lineages. Endodermal lineage: DMEM low glucose, 10% FCS and 2 mM L -glutamine and penicillin/streptomycin. Mesodermal lineage: IMDM, 20% FCS, 2 mM L -glutamine and penicillin/streptomycin, 1% nonessential amino acids, 0.05 mM β-mercaptoethanol and 0.004% ALPHA-thioglycerol (Sigma Aldrich). Ectodermal lineage: N2B27 medium without retinoic acid, supplemented with 5 μM SB431542 activin A receptor inhibitor (Sigma Aldrich). Accession codes: Global gene expression analysis and microarray data processing were performed as previously described [42] . Microarray data are accessible via the GEO (Gene Expression Omnibus) website under accession number GSE21302 . How to cite this article: Tapia, N. et al. Reprogramming to pluripotency is an ancient trait of vertebrate Oct4 and Pou2 proteins. Nat. Commun. 3:1279 doi: 10.1038/ncomms2229 (2012).